Mia40 targets cysteines in a hydrophobic environment to direct oxidative protein folding in the mitochondria Mia40 catalyses the oxidative folding of disulphide-containing proteins in the mitochondria. The folding pathway is directed by the formation of the first mixed disulphide between Mia40 and its substrate. Here, we employ Cox17 to elucidate the molecular determinants of this reaction. Mia40 engages initially in a dynamic non-covalent enzyme–substrate complex that forms and dissociates within milliseconds. Cys36 of Cox17 forms the mixed disulphide in an extremely rapid reaction that is limited by the preceding complex formation with Mia40. Cys36 reacts much faster than the three other cysteines of Cox17, because it neighbours three hydrophobic residues. Mia40 binds preferentially to hydrophobic regions and the dynamic nature of the non-covalent complex allows rapid reorientation for an optimal positioning of the reactive cysteine. Mia40 thus uses the unique proximity between its substrate-binding site and the catalytic disulphide to select a particular cysteine for forming the critical initial mixed disulphide. The intermembrane space (IMS) of the mitochondria was long believed to provide a reducing environment, similar to the cytosol, but recently proteins with disulphide bonds and subsequently a thiol oxidase (Mia40, mitochondrial import and assembly) were discovered in the IMS [1] , [2] , [3] , [4] , [5] , [6] , [7] , [8] , [9] , [10] , [11] , [12] . Unlike the other known thiol oxidases, Mia40 does not belong to the thioredoxin family, and its catalytic disulphide is arranged in a unique Cys-Pro-Cys motif. The catalytic domain consists of two antiparallel α helices [13] , [14] ( Fig. 1a,b ). They form a shallow hydrophobic groove, which is believed to bind protein substrates in a helical conformation [13] , [14] , [15] . 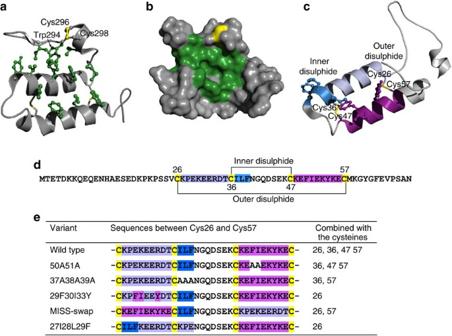Figure 1: Structures of Mia40 and Cox17. (a) Backbone structure of Mia40 fromS.cerevisiae. Sulphur atoms of the catalytic disulphide are coloured yellow, residues of the hydrophobic groove are coloured green. Residues are numbered according to the amino-acid sequence of full-length Mia40. (b) Surface representation of Mia40, colouring and orientation is as in (a). Panelsaandbwere created using Protein Data Bank files 2ZXT (Mia40)14and IU97 (Cox17)17and the programme PyMOL. (c) Backbone structure of Cox17 fromS.cerevisiae. Sulphur atoms of the structural disulphides are coloured yellow, cysteines are numbered according to the amino-acid sequence. The first CX9C motif is coloured purple (residues 26–33), the second CX9C motif (residues 47–57) is magenta and the hydrophobic residues 37–39 following Cys36 are blue. The residues of the MISS/ITS sequence (F50, I51, Y54) and I37, L38, F39 are shown in ball and sticks representation. (d) Amino-acid sequence of Cox17 fromS.cerevisiae. Cys16, Cys23 and Cys24 that bind Cu2+were substituted by Ser in all variants used here. Structural cysteines are highlighted yellow and the native disulphide bonds are indicated. Residues were coloured according to the structure in (c). (e) Summary of the variants that were used to analyse the reactivity of single-cysteine variants of Cox17*. The sequences encompassing the two CX9C motifs (in pale blue and magenta, respectively) are depicted. The ILF motif after C36 is shown in blue; cysteines are shown in yellow. The sequences in the middle were combined with single cysteines as indicated in the right column and used for following mixed disulphide formation or for producing the AEDANS-labelled variants for the binding studies. A numbered list of all 33 variants is provided inSupplementary Table S1. Figure 1: Structures of Mia40 and Cox17. ( a ) Backbone structure of Mia40 from S . cerevisiae . Sulphur atoms of the catalytic disulphide are coloured yellow, residues of the hydrophobic groove are coloured green. Residues are numbered according to the amino-acid sequence of full-length Mia40. ( b ) Surface representation of Mia40, colouring and orientation is as in ( a ). Panels a and b were created using Protein Data Bank files 2ZXT (Mia40) [14] and IU97 (Cox17) [17] and the programme PyMOL. ( c ) Backbone structure of Cox17 from S . cerevisiae . Sulphur atoms of the structural disulphides are coloured yellow, cysteines are numbered according to the amino-acid sequence. The first CX 9 C motif is coloured purple (residues 26–33), the second CX 9 C motif (residues 47–57) is magenta and the hydrophobic residues 37–39 following Cys36 are blue. The residues of the MISS/ITS sequence (F50, I51, Y54) and I37, L38, F39 are shown in ball and sticks representation. ( d ) Amino-acid sequence of Cox17 from S . cerevisiae . Cys16, Cys23 and Cys24 that bind Cu 2+ were substituted by Ser in all variants used here. Structural cysteines are highlighted yellow and the native disulphide bonds are indicated. Residues were coloured according to the structure in ( c ). ( e ) Summary of the variants that were used to analyse the reactivity of single-cysteine variants of Cox17*. The sequences encompassing the two CX 9 C motifs (in pale blue and magenta, respectively) are depicted. The ILF motif after C36 is shown in blue; cysteines are shown in yellow. The sequences in the middle were combined with single cysteines as indicated in the right column and used for following mixed disulphide formation or for producing the AEDANS-labelled variants for the binding studies. A numbered list of all 33 variants is provided in Supplementary Table S1 . Full size image Most, but not all, substrates of Mia40, belong to the families of CX 9 C and CX 3 C proteins [3] , [11] , [16] . Similar to Mia40 itself, these proteins are composed of two short antiparallel helices that are covalently linked by two disulphide bonds. This is shown for the CX 9 C protein Cox17 (ref. 17 ) in Fig. 1c,d . Here the two helices are linked by the two structural disulphide bonds Cys36-Cys47 (the inner disulphide) and Cys26-Cys57 (the outer disulphide). Enzyme-catalysed oxidative folding in other compartments such as the bacterial periplasm or the ER is well understood [4] , [18] , [19] , [20] , [21] . It involves complex systems of thiol-disulphide oxidoreductases that use thioredoxin-like domains for introducing disulphides into folding protein chains and for isomerizing incorrect disulphides that form preferentially early in folding. Oxidative folding mediated by Mia40 appears to differ from these principles, and two cases can be envisioned for how Mia40 might function. Similar to the enzymes in the ER and the periplasm, it might first introduce random, mostly local disulphide bonds, and then correct them by catalysing isomerization reactions. Alternatively, Mia40 might be able to interact preferentially with certain cysteine residues to direct the folding pathway of its substrate towards the formation of the correct disulphide bonds and to avoid the necessity of disulphide isomerizations. In the ‘sliding-and-docking’ model for the mechanism of Mia40, it was proposed that Mia40 uses the amphipathic character of one of the helices formed in the substrate protein to steer the oxidation mechanism [22] , [23] . Hydrophobic residues that are one and/or two turns away from a cysteine residue in the helix form a so-called MISS (mitochondrial IMS sorting signal) [24] or ITS (IMS targeting signal) [22] motif. Its binding to the hydrophobic surface of Mia40 was assumed to position a particular cysteine to form the critical first mixed disulphide. In the case of Cox17, the second helix was suggested to contain the MISS/ITS motif and Cys45 of human Cox17 or Cys57 of yeast Cox17 to form the initial mixed disulphide. Accordingly, the outer disulphide bond was assumed to form first in yeast Cox17, the inner disulphide in human Cox17 (ref. 22 ). This model could not explain how the other disulphide is formed in the yeast protein [23] , [25] , because the MISS/ITS sequence would be no longer accessible for a second reaction with Mia40. The formation of the initial mixed disulphide between Mia40 and a substrate protein directs the course of its oxidative folding [23] . Here, we use a kinetic analysis and sequence variants of yeast Cox17 and Mia40 to dissect the individual steps of this reaction and to examine how they are determined by the environment of the reacting cysteine residues. In particular, we find that Cys36 reacts much faster with Mia40 than all other Cys residues, favoring introduction of the inner disulphide of Cox17 first. We arrive at a simple model in which Mia40 kinetically selects cysteines neighboured by hydrophobic residues for forming the initial enzyme–substrate-mixed disulphide as the decisive initial reaction intermediate. Unfolded proteins bind to Mia40 in a highly dynamic reaction Catalysed oxidative folding involves thiol/disulphide exchange reactions that follow general mechanisms, irrespective of the nature of the thiol oxidase. The reaction starts with the non-covalent binding of the protein substrate to the thiol oxidase, followed by the formation of the mixed disulphide. This mixed disulphide is then resolved either by the back reaction in which the second Cys of the thiol oxidase displaces the substrate protein or by the attack of another cysteine of the substrate protein. Equation (1) provides a kinetic scheme for initial non-covalent complex formation and subsequent mixed disulphide formation between Mia40 and Cox17 variants with single cysteines. We employed Förster resonance energy transfer (FRET) to investigate how yeast Mia40 forms the initial complex with Cox17 and to determine its lifetime. All variants of Cox17 contained only the four structural cysteine residues of the twin CX 9 C motif. The cysteines 16, 23 and 24 of the Cu 2+ binding site were replaced by serines. We label the corresponding pseudo wild-type protein as Cox17*. Figure 1e provides an overview of the Cox17 variants that were used to analyse binding and mixed disulphide formation. A numbered list of all variants is given in Supplementary Table S1 . To uncouple non-covalent binding from the subsequent formation of the mixed disulphide, a variant of Mia40 (Aed-Mia40) without the Cys296-Cys298 active-site disulphide was employed. Cys298 was substituted by Ser, and Cys296 was modified covalently with AEDANS, to serve as an acceptor of energy transferred from a tryptophan in the substrate protein. Wild-type Cox17 is devoid of Trp, and therefore a Trp was introduced by the F50W substitution. The single Trp of Mia40 was removed by the W294F replacement. Binding of Cox17* F50W to Aed-Mia40 thus could be followed by the increase in AEDANS fluorescence after the excitation of Cox17* F50W. The 1–25 region of Cox17 is polar and unfolded, the remainder (26–69) contains the two helices that are linked by the disulphide bonds ( Fig. 1c ). The amide CD spectrum of Cox17* reflects this mixture of helical and random-coil segments ( Supplementary Fig. S1a ). Folded Cox17* with intact disulphide bonds is not bound by Aed-Mia40 ( Supplementary Fig. S2a ), presumably because it does not expose sufficient hydrophobic surface. Reduced Cox17* F50W is unfolded ( Supplementary Fig. S1a ). It is bound by Aed-Mia40 with high affinity, and the titration followed by FRET ( Supplementary Fig. S2b ) gave a K D value of 4.8 μM ( Table 1 ). This binding reaction is extremely rapid. In the presence of 10 μM Cox17* F50W, it shows an apparent rate constant of 140 s −1 and is almost complete within 20 ms ( Fig. 2a ). As expected for a simple association reaction, the measured rate constant increases linearly with Cox17* F50W concentration ( Fig. 2b ). The analysis gives an association rate k on =9.5 s −1 μM −1 from the slope and a dissociation rate k off =43 s −1 from the intercept ( Table 1 ), which is equivalent to an average lifetime of only 23 ms, indicating that the complex between Mia40 and reduced Cox17* is extremely dynamic. The ratio k off / k on is a reliable measure of the equilibrium constant. Its value of 4.6 μM ( Table 1 ) is similar to the value of 4.8 μM, as obtained from the titration curve ( Supplementary Fig. S2b ). The analysis of the amplitudes of association ( Fig. 2c ) gave a K D value of 2.6 μM. Reduced Cox17* F50W thus interacts with Mia40 with micromolar affinity in an extremely dynamic binding reaction. Table 1 Association of Mia40 with Cox17* and mixed disulphide formation. 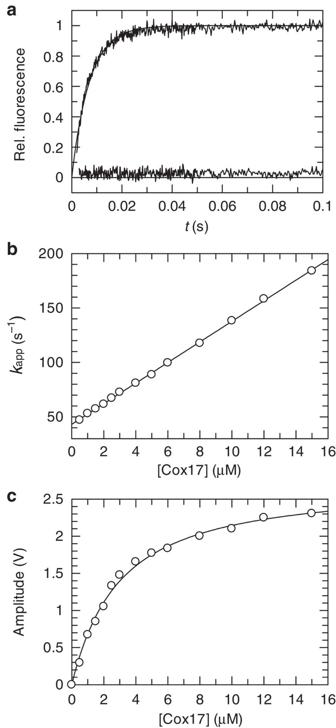Figure 2: Complex formation between Aed-Mia40 and Cox17* F50W. (a) Time course of association between 0.5 μM Aed-Mia40 and 0 or 10 μM reduced Cox17* F50W (variant 1). Data were analysed with monoexponential functions. (b) Dependence of the measured rate constants and (c) dependence of the amplitudes of complex formation on the concentration of reduced Cox17*F50W. Values forkoffandkonwere derived from the intercept and the slope of the line in (b), respectively. Amplitudes were analysed assuming a simple 1:1 binding reaction. The kinetics was followed by fluorescence above 450 nm after excitation at 280 nm. All measurements were performed in 0.1 M potassium phosphate, 1 mM EDTA, pH 7.4 at 15 °C. All values derived from the analysis of the data are given inTable 1. Full size table Figure 2: Complex formation between Aed-Mia40 and Cox17* F50W. ( a ) Time course of association between 0.5 μM Aed-Mia40 and 0 or 10 μM reduced Cox17* F50W (variant 1). Data were analysed with monoexponential functions. ( b ) Dependence of the measured rate constants and ( c ) dependence of the amplitudes of complex formation on the concentration of reduced Cox17*F50W. Values for k off and k on were derived from the intercept and the slope of the line in ( b ), respectively. Amplitudes were analysed assuming a simple 1:1 binding reaction. The kinetics was followed by fluorescence above 450 nm after excitation at 280 nm. All measurements were performed in 0.1 M potassium phosphate, 1 mM EDTA, pH 7.4 at 15 °C. All values derived from the analysis of the data are given in Table 1 . Full size image A variant with the inner (C36-C47) disulphide bond only (Cox17*-innerSS, variant 2) was produced by the C26A, C57S replacements, a variant with the outer (C26-C57) disulphide bond only (Cox17*-outerSS, variant 3) by the C36I, C47A substitutions. The CD spectrum of the variant with the inner disulphide bond intact lies between the spectra of the reduced and oxidized forms of Cox17* ( Supplementary Fig. S1a ), indicating that Cox17*-innerSS is partially unfolded. The variant with the outer disulphide is largely folded, suggesting that its formation is sufficient for Cox17* to adopt an ordered structure ( Supplementary Fig. S1a ). However, measurement of the CD as a function of temperature ( Supplementary Fig. S1b ) reveals that Cox17*-outerSS is strongly destabilized relative to the wild-type protein with both disulphides intact. Cox17*-innerSS is half-unfolded at 10 °C. For Cox17*-outerSS, binding could neither be detected at equilibrium ( Supplementary Fig. S2a ) nor in a kinetic experiment ( Supplementary Fig. S3a ), presumably because its native-like conformation impairs the interaction with Mia40. After formation of the inner disulphide bond, Cox17* is still accessible for Aed-Mia40, but binding is weak ( Supplementary Fig. S2a ). The rate of its association with Aed-Mia40 ( Supplementary Fig. S3b ) is more than twofold decreased and the rate of dissociation twofold increased ( Table 1 ), leading to a fivefold increase in k off / k on . After reduction, both single-disulphide variants of Cox17* became unfolded and interacted with Aed-Mia40 in a similar fashion as reduced Cox17* F50W ( Table 1 ). A combined variant with all four cysteines substituted was produced as well (Cox17*-0Cys, variants 6 and 7). It is unfolded ( Supplementary Fig. S1a ), and, similar to the other variants without disulphides, it associated with Aed-Mia40 rapidly with an association rate near 9 s −1 μM −1 and a K D of 11.7 μM ( Table 1 ). The affinity and the kinetics of binding of Mia40 to its substrate protein thus correlate with the extent of unfolding. Variants of Cox17* without disulphide bonds or with only the inner disulphide are substrates for Mia40, the forms with the native disulphides or with the outer disulphide are folded and thus not substrates for Mia40. Labelling exerts only a small effect on the binding kinetics In Aed-Mia40, the AEDANS group is linked to Cys296 close to the presumed binding site for unfolded protein chains ( Fig. 1a ). To examine whether this modification influenced binding, we performed experiments in which the energy donor Trp was placed in Mia40 and the acceptor AEDANS in Cox17*. Four single-cysteine variants of Cox17* were produced and labelled with AEDANS (variants 8–11). Their interaction with the wild-type form of Mia40 was then measured in equilibrium titrations, and its kinetics was followed in the stopped-flow instrument by the FRET between the single Trp (W294) of Mia40 and the AEDANS groups of the four Cox17* variants ( Supplementary Fig. S4 ). The position of the label has a small influence on the measured K D values and rates of association and dissociation, but the very high dynamics of substrate binding and dissociation is conserved ( Table 1 ). The energy transfer upon binding was very small when the AEDANS label was bound to Cys26 ( Supplementary Fig. S4b ), possibly because Cys26 is remote from the donor Trp294, which resides near the active site of Mia40 ( Fig. 1 ). Mia40 shows generic binding to unfolded proteins. α-lactalbumin is a small milk protein with four disulphide bonds that matures in the ER. It unfolds after reduction and carboxymethylation, and it binds to Aed-Mia40 as rapidly as the Cox17* variants ( k on =13 s −1 μM −1 , Table 1 ). The complex is also short-lived and shows a lifetime of only 4 ms. Apparently, highly dynamic binding is an intrinsic property of Mia40. It is also observed for an unrelated unfolded protein and not limited to dedicated substrates with potential recognition motifs. Cys of Cox17* differ in mixed disulphide formation with Mia40 After non-covalent binding, Mia40 and its substrate protein form a covalent mixed disulphide (Equation (1)). To examine its formation, we employed the four variants of Cox17* with only a single cysteine (variants 12–15). Their mixed disulphides with Mia40 accumulate, because they cannot be resolved by another cysteine of the substrate. Only the reversal of their formation is possible ( k −2 , Equation (1)). Formation of the mixed disulphides was initiated by mixing 20 μM each of Mia40 and of the single-Cys variants of Cox17*. After 5 s and 5 min, respectively, the thiol-disulphide exchange reaction was stopped by adding iodoacetate, and the samples were subjected to SDS–PAGE ( Fig. 3a ). The three Cox17* variants with the cysteines 36, 47 and 57 reacted very rapidly with Mia40, and the mixed disulphide was formed essentially within 5 s. The variant with Cys26 reacted more slowly. All mixed disulphides appeared to be stable for 5 min, and they were reduced by dithiothreitol (DTT), as expected for intermolecular disulphide bonds ( Fig. 3a ). 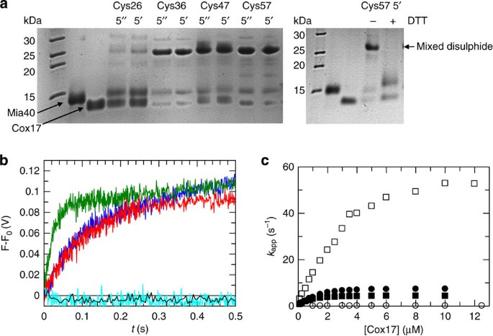Figure 3: Formation of the mixed disulphide between Mia40 and Cox17*. (a) Left, 20 μM Mia40 and 20 μM of the single-cysteine variants of Cox17* (variants 12–15) were co-incubated, and after 5 s and 5 min, respectively, the reaction was stopped by adding iodoacetate. Right, the mixed disulphide with Cys57, as present after 5 min, is cleaved by DTT. The samples were analysed by SDS–PAGE. (b) 0.25 μM Mia40 and 6 μM Cox17* 26C (black), Cox17* 36C (green), Cox17* 47C (blue) and Cox17* 57C (red), respectively, were mixed and the increase in fluorescence above 320 nm (F) upon complex formation is shown as a function of time. The initial fluorescence (F0) was subtracted. As a control, the reaction between 0.25 μM Mia40 and 6 μM Cox17*-0Cys (variant 6) (cyan) was measured as well. Data were analysed with monoexponential functions with a linear term. (c) The rate constants of the reaction between 0.25 μM Mia40 and Cox17* 26C (open circles), Cox17* 36C (open squares), Cox17* 47C (filled squares) and Cox17* 57C (filled circles) are shown. All measurements were performed in 0.1 M potassium phosphate, 1 mM EDTA, pH 7.4 at 15 °C. Figure 3: Formation of the mixed disulphide between Mia40 and Cox17*. ( a ) Left, 20 μM Mia40 and 20 μM of the single-cysteine variants of Cox17* (variants 12–15) were co-incubated, and after 5 s and 5 min, respectively, the reaction was stopped by adding iodoacetate. Right, the mixed disulphide with Cys57, as present after 5 min, is cleaved by DTT. The samples were analysed by SDS–PAGE. ( b ) 0.25 μM Mia40 and 6 μM Cox17* 26C (black), Cox17* 36C (green), Cox17* 47C (blue) and Cox17* 57C (red), respectively, were mixed and the increase in fluorescence above 320 nm ( F ) upon complex formation is shown as a function of time. The initial fluorescence ( F 0 ) was subtracted. As a control, the reaction between 0.25 μM Mia40 and 6 μM Cox17*-0Cys (variant 6) (cyan) was measured as well. Data were analysed with monoexponential functions with a linear term. ( c ) The rate constants of the reaction between 0.25 μM Mia40 and Cox17* 26C (open circles), Cox17* 36C (open squares), Cox17* 47C (filled squares) and Cox17* 57C (filled circles) are shown. All measurements were performed in 0.1 M potassium phosphate, 1 mM EDTA, pH 7.4 at 15 °C. Full size image Since mixed disulphide formation between Mia40 and the single-Cys variants of Cox17* is so fast, manual mixing and chemical quenching with iodoacetate were not suitable for following its kinetics. It could be followed, however, by the fluorescence of Mia40, which is sensitive to reduction of the catalytic disulphide bond. This could be shown via reduction with GSH. The fluorescence increases about threefold upon reduction with GSH ( Supplementary Fig. S5a ) in a two-step reaction ( Supplementary Fig. S5b ). Both mixed disulphide formation (rate constant=8 s −1 M −1 , Supplementary Fig. S5c ) and its resolution by a second GSH molecule (rate constant=0.6 s −1 M −1 ) led to strong increases in fluorescence, as observed previously by Banci et al. [13] for human Mia40. A similar increase in fluorescence upon reduction has also been observed for DsbA of E . coli . In the oxidized form, the catalytic disulphide probably quenches Trp emission and this quenching is relieved upon reduction. The fluorescence of Mia40 increased also when the mixed disulphides with the single-Cys variants of Cox17* were formed. 6 μM of the single-Cys variants of Cox17* were mixed rapidly with 0.25 μM Mia40 in a stopped-flow apparatus ( Fig. 3b ). The reaction of Cys36 with Mia40 was extremely fast and virtually complete in 100 ms. The reactions with Cys47 and Cys57 were slower and required about 1 s for completion, whereas Cys26 reacted with Mia40 so slowly that little fluorescence change could be observed within the time range of the stopped-flow experiment. Formation of the mixed disulphide was followed by a slow phase. Its rate was strongly pH-dependent, but independent of the concentrations of Mia40 and Cox17*, which suggests that it involves a slow intramolecular thiol-disulphide exchange reaction, possibly transfer to the second active site Cys of Mia40. The fluorescence did not increase when Mia40 was mixed with the cysteine-free variant Cox17*-0Cys ( Fig. 3b ). In subsequent experiments, the Mia40 concentration was held constant at 0.25 μM, and the concentrations of the single-Cys variants of Cox17* were varied between 0 and 12 μM ( Fig. 3c ). Initially, the measured pseudo first-order rate increased linearly with Cox17* concentration, which indicates that, under these conditions, mixed disulphide formation is limited by the association between Mia40 and the Cox17* variants. For the interaction of Mia40 with Cys36 of Cox17*, we observed an initial slope of 12 s −1 μM −1 , which agrees well with the rate constant of the non-covalent association between Mia40 and reduced Cox17*, which is near 10 s −1 μM −1 ( Table 1 ). This is remarkable, because it indicates that mixed disulphide formation between Cys36 of Cox17* and Mia40 in the bound state is so fast that it is limited in rate by the preceding very rapid non-covalent association reaction. It is also 10 6 -fold faster than the corresponding reaction with GSH ( Supplementary Fig. S5c ). With increasing Cox17* concentration, saturation behaviour is observed, and above 10 μM of the Cox17* variants, the rates of mixed disulphide formation become constant ( Fig. 3c ). At these high concentrations, association is very fast, and the rate-limiting step shifts from association to mixed disulphide formation in the complex. Rate profiles such as those in Fig. 3a are typical for kinetic two-step mechanisms (Equation (1)) in which a binding reaction is followed by an isomerization, in our case, by the formation of the mixed disulphide. The initial slope usually reflects the second-order rate of the association reaction ( k on ), and the limiting value for the apparent rate of the second step at high ligand concentration reflects k 2 + k −2 (Equation (1)). At 10 μM Cox17*, we observed huge differences in the rates of mixed disulphide formation. Cys36 reacts extremely fast with Mia40 and shows an apparent rate of 53 s −1 . With apparent rates of 4.3 s −1 and 9.8 s −1 , respectively, Cys47 and Cys57 react 5–10-fold more slowly than Cys36. This is unexpected since Cys45 of human Cox17 and Cys57 of yeast Cox17 were suggested to form the initial mixed disulphide with Mia40, because they flank the MISS/ITS sequence [15] , [26] . Cys26 is almost nonreactive in the Mia40-bound state. With a rate constant of 0.12 s −1 , it forms the mixed disulphide 400-fold more slowly than Cys36 ( Fig. 3c ). All single-cysteine variants are unfolded, and therefore the differences in reactivity do not originate from differences in accessibility. The individual cysteines of Cox17* differ also in the fluorescence increases that accompany mixed disulphide formation with Mia40. The cysteines 36, 47 and 57 show large amplitudes (70–90 fluorescence units at 10 μM Cox17*, Table 1 ), presumably because the mixed disulphides form readily and are stable at equilibrium. The reaction with Cys26 led to an increase by only 8 fluorescence units ( Table 1 ), confirming that Cys26 forms the mixed disulphide to a small extent only (cf. Fig. 3a ). The Cys reactivities are not determined by their p K values The formation of the mixed disulphide involves the nucleophilic attack of the catalytic disulphide of Mia40 by a substrate thiolate anion. Consequently, its rate depends on the relative concentration of the deprotonated form of the respective cysteine, and thus on its pK value. The rates of mixed disulphide formation under saturation conditions (15 μM Cox17*, variants 12–15) measured as a function of pH ( Fig. 4 ) follow the titration curves of the individual cysteine residues. They give apparent pK values that range between 7.0 (for Cys36) and 8.2 (for Cys26). The Brønsted coefficient for thiol/disulphide exchange reactions is about 0.5 (ref. 27 ), and therefore a fourfold difference in reactivity would be expected between Cys26 and Cys36. The observed 400-fold difference is thus not explained by the difference in pK. Moreover, the reaction rates remain to be strongly different at pH 9 (50-fold between Cys26 and Cys36), conditions under which the thiolate form predominates for all four Cys residues. 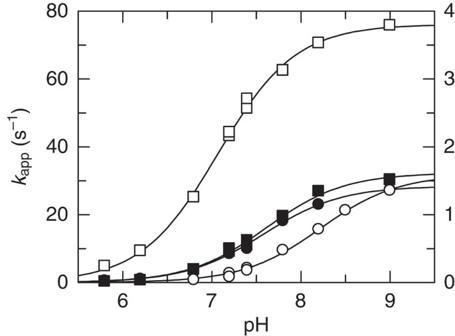Figure 4: Ionization properties of the cysteines of Cox17*. 0.25 μM Mia40 was mixed with 15 μM Cox17* 26C (open circles), Cox17* 36C (open squares), Cox17* 47C (filled squares) and Cox17* 57C (filled circles), respectively, (variants 12–15) and the increase in fluorescence above 320 nm after excitation at 280 nm was detected. The fluorescence traces were analysed with monoexponential functions with a linear term, and the rate constants (kapp) are plotted as a function of pH. Data points for Cox17* 26C refer to the right ordinate. Apparent pK values were determined with the Henderson–Hasselbalch equation to be 8.2 for Cys26, 7.0 for Cys36, 7.6 for Cys47 and 7.7 for Cys57. Measurements were performed at 15 °C in 0.1 M potassium phosphate (pH 5.8, 6.2, 6.8, 7.2 and 7.4) or 0.1 M Tris–HCl (pH 7.2, 7.4, 7.8, 8.2 8.5 and 9.0). Figure 4: Ionization properties of the cysteines of Cox17*. 0.25 μM Mia40 was mixed with 15 μM Cox17* 26C (open circles), Cox17* 36C (open squares), Cox17* 47C (filled squares) and Cox17* 57C (filled circles), respectively, (variants 12–15) and the increase in fluorescence above 320 nm after excitation at 280 nm was detected. The fluorescence traces were analysed with monoexponential functions with a linear term, and the rate constants ( k app ) are plotted as a function of pH. Data points for Cox17* 26C refer to the right ordinate. Apparent pK values were determined with the Henderson–Hasselbalch equation to be 8.2 for Cys26, 7.0 for Cys36, 7.6 for Cys47 and 7.7 for Cys57. Measurements were performed at 15 °C in 0.1 M potassium phosphate (pH 5.8, 6.2, 6.8, 7.2 and 7.4) or 0.1 M Tris–HCl (pH 7.2, 7.4, 7.8, 8.2 8.5 and 9.0). Full size image The four Cys residues of Cox17* thus show huge differences in reactivity that are not explained by differences in accessibility or chemical reactivity. We suggest that the rate of mixed disulphide formation is determined by the average distance between the cysteines and the catalytic disulphide of Mia40 in the initial non-covalent complex. Interestingly, a very small energy transfer was observed between Cox17* and Mia40 ( Supplementary Fig. S4b,c ), when the AEDANS label was linked to Cys26. This also indicates that in the non-covalent complex Cys26 is remote from the active site of Mia40. MISS/ITS influences complex formation of Mia40 with Cox17 The current sliding-and-docking model assumes that substrate proteins bind to Mia40 in a helical conformation and that the hydrophobic residues of a MISS/ITS sequence 3, 4 and 7 positions apart from a cysteine are essential for docking and orienting this cysteine for rapid reaction with the catalytic disulphide of Mia40. In Cox17, the MISS/ITS sequence is located between Cys47 and Cys57. Binding to this sequence should thus favour mixed disulphide formation with one of these two cysteines, and not with Cys36, as observed experimentally. The central positions of the MISS/ITS sequence of Cox17 are occupied by Phe50 and Ile51. The substitutions of both by Ala in the three Cox17* variants with single cysteines at the positions 36, 47 or 57 (variants 16–18) led to 20–60-fold decreases in the rate of association ( k on ) with Mia40 ( Supplementary Fig. S6 ), and corresponding decreases in affinity ( k off / k on , Table 1 ). These two hydrophobic residues are thus of general importance for the non-covalent binding of unfolded forms of Cox17* to Mia40 in step 1 of Equation (1). In contrast, the effects on the kinetics of mixed disulphide formation (employing variants 19–21) after binding ( Fig. 5 ) were small and not restricted to Cys47 and Cys57 that flank the MISS/ITS sequence. The rate of this reaction was fivefold decreased for Cys57 ( Fig. 5d ), 2.5-fold decreased for Cys47 ( Fig. 5c ) and still twofold decreased for Cys36 ( Fig. 5b ), which is remote from the MISS/ITS sequence. The rates observed at 10 μM of the Cox17* variants are shown in Table 1 , Supplementary Fig. S7 depicts the corresponding amplitudes. Together, this suggests that the MISS/ITS residues enhance the rate of initial complex formation (step 1, Equation (1)), but seem to be less important for selecting a cysteine of the substrate protein to form the first mixed disulphide in the second step of Equation (1). 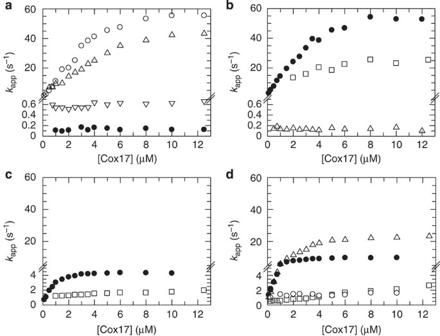Figure 5: Kinetics of mixed disulphide formation between Mia40 and Cox17* variants. Mixed disulphide formation between 0.25 μM Mia40 and increasing concentrations of the Cox17* variants was followed by the increase in fluorescence above 320 nm. The rate constants are shown for (a) Cox17* 26C, variant 12 (filled circles), Cox17* 26C 27I28L29F, variant 32 (open triangles), Cox17* 26C 29F30I33Y, variant 27 (inverted triangles), Cox17* 26C-MISS-swap, variant 30 (open circles). (b) Cox17* 36C, variant 13 (filled circles), Cox17* 36C 37A38A39A, variant 23 (open triangles), Cox17* 36C 50A51A, variant 19 (open squares). (c) Cox17* 47C, variant 14 (filled circles), Cox17* 47C 50A51A, variant 20 (open squares). (d) Cox17* 57C, variant 15 (filled circles), Cox17* 57C 50A51A, variant 21 (open squares), Cox17* 57C 37A38A39A, variant 23 (open triangles), Cox17* 57C MISS-swap, variant 31 (open circles). Data were analysed with monoexponential functions with a linear term. The corresponding amplitudes are shown inSupplementary Fig. S7. All measurements were performed in 0.1 M potassium phosphate, 1 mM EDTA, pH 7.4 at 15 °C. Figure 5: Kinetics of mixed disulphide formation between Mia40 and Cox17* variants. Mixed disulphide formation between 0.25 μM Mia40 and increasing concentrations of the Cox17* variants was followed by the increase in fluorescence above 320 nm. The rate constants are shown for ( a ) Cox17* 26C, variant 12 (filled circles), Cox17* 26C 27I28L29F, variant 32 (open triangles), Cox17* 26C 29F30I33Y, variant 27 (inverted triangles), Cox17* 26C-MISS-swap, variant 30 (open circles). ( b ) Cox17* 36C, variant 13 (filled circles), Cox17* 36C 37A38A39A, variant 23 (open triangles), Cox17* 36C 50A51A, variant 19 (open squares). ( c ) Cox17* 47C, variant 14 (filled circles), Cox17* 47C 50A51A, variant 20 (open squares). ( d ) Cox17* 57C, variant 15 (filled circles), Cox17* 57C 50A51A, variant 21 (open squares), Cox17* 57C 37A38A39A, variant 23 (open triangles), Cox17* 57C MISS-swap, variant 31 (open circles). Data were analysed with monoexponential functions with a linear term. The corresponding amplitudes are shown in Supplementary Fig. S7 . All measurements were performed in 0.1 M potassium phosphate, 1 mM EDTA, pH 7.4 at 15 °C. Full size image Adjacent hydrophobic residues boost the reactivity of Cys36 The catalytic disulphide of Mia40 and the hydrophobic binding groove are close to each other ( Fig. 1a,b ). The reactivity of a particular cysteine might therefore depend on the presence of hydrophobic residues in its immediate vicinity. Cys36 is followed by three non-polar residues: Ile37, Leu38 and Phe 39 ( Fig. 1c,d ). The substitution of these three residues by Ala (in Cox17* 36C 37A38A39A, variants 22 and 23), reduced the affinity ( k off / k on ) about tenfold ( Supplementary Fig. S8d ), mostly because k off was increased ( Table 1 ). Interestingly, the amplitude of binding was also reduced ( Supplementary Fig. S8c ), suggesting that in the complex with this variant of Cox17*, the AEDANS-labelled Cys36 is shifted to a position further remote from Trp294 of Mia40, which resides near the catalytic disulphide. The substitution of the three hydrophobic residues after Cys36 led to an about 400-fold deceleration of the mixed disulphide formation ( Fig. 5b ), and with a rate of 0.17 s −1 , Cys36 now reacted as slowly as Cys26, which is the least reactive cysteine of Cox17* ( Table 1 ). The three hydrophobic residues at the positions 37–39 were also substituted in the variant with the single cysteine at position 57 (Cox17* 57C 37A38A39A, variants 24 and 25). Interestingly, its rate of mixed disulphide formation increased from 9.8 s −1 to 22.5 s −1 . This also suggests that in Cox17*, residues Ile37, Leu38, and Phe39 bind close to the active site, which disfavours mixed disulphide formation with the remote Cys57. We conclude that the unusually high rate of the thiol-disulphide exchange reaction between Cys36 of Cox17* and the catalytic disulphide of Mia40 is caused by the preferential interaction of Ile37, Leu38, and Phe39 with the hydrophobic binding surface of Mia40. This binding directs Cys36 to a position very close to the catalytic disulphide of Mia40 and thus increases its effective concentration for mixed disulphide formation several hundred fold. Apparently, the three hydrophobic residues after Cys36 are much more efficient in directing initial disulphide formation than the MISS/ITS sequence. Cys26 is activated by introducing hydrophobic residues To examine whether the very low reactivity of Cys26 could be improved by modulating the sequence in its environment, we first inserted three residues of the MISS/ITS sequence as present after Cys 47 (Phe50, Ile51 and Tyr54) at the equivalent positions after Cys26 (by the substitutions E29F, K30I and R33Y, variants 26 and 27). This led to an about twofold increase in the rate of association ( k on ) and in affinity ( Supplementary Fig. S8b , Table 1 ). The very low reactivity of Cys26 towards thiol-disulphide exchange with Mia40 was about sixfold increased ( Fig. 5a ) but remained still 10-fold lower than the reactivities of Cys47 and Cys57 and 150-fold lower than the reactivity of Cys36 ( Table 1 ). The E29F K30I R33Y variant contains two MISS/ITS sequences, the original one between Cys47 and Cys57 and the engineered one between Cys 26 and Cys 36, and they might compete with each other. We therefore exchanged the entire sequence between Cys26 and Cys36 of the fist CX 9 C motif with the sequence between Cys47 and Cys57 of the second CX 9 C motif (that contains the MISS/ITS sequence). The MISS/ITS sequence was thus moved from the vicinity of Cys57 to the vicinity of Cys26 in the two variants that contain Cys26 and Cys57, respectively (variants 28–31). They were first labelled with AEDANS to measure the kinetics of non-covalent binding to Mia40. In both cases, the dynamics of binding and the affinity ( k off / k on ) were changed to a small extent only by the swapping of the sequences of the two CX 9 C motifs ( Supplementary Fig. S8a,b,g,h ). Presumably, the overall hydrophobicity of unfolded Cox17 is an important factor for binding, and this is not changed in the sequence-swapped variants. A strong difference was observed, however, for the amplitudes of association. After sequence swapping, the amplitude was 20-fold reduced when the acceptor AEDANS was attached to Cys57 ( Supplementary Fig. S8g ) and 20-fold increased when attached to Cys26 ( Supplementary Fig. S8a ). The amplitude of binding depends among other factors on the average distance between Trp294 near the active site of Mia40 and the AEDANS group on the cysteine of the substrate protein. The 20-fold changes in the binding amplitudes thus suggest that in the sequence-swapped protein, the mode of binding has changed. Unlike in the wild-type protein, Cys26 now seems to be much closer to the active site of Mia40 than Cys57. The shift of the MISS/ITS sequence away from the vicinity of Cys57 to the vicinity of Cys26 had a profound effect on mixed disulphide formation with Mia40. Its rate decreased sixfold for Cys57 ( Fig. 5d ), and, at the same time, it was 400-fold increased for Cys26 ( Fig. 5a , Table 1 ). The 400-fold decrease in the reactivity observed for Cys36 in a variant in which the residues Ile37, Leu38 and Phe39 were replaced by alanines ( Table 1 ) indicated that these three hydrophobic residues are responsible for the unusually high reactivity of Cys36. We now asked whether they would also activate Cys26 for mixed disulphide formation with Mia40. To this end, we shifted the residues Ile, Leu and Phe from the positions 37–39 after Cys36 to 27–29 after Cys26 and reciprocally Lys, Pro and Glu from the positions 27–29 to 37–39 (variants 32 and 33). For this variant (Cox17* 27I 28L 29F), the rate of mixed disulphide formation of Cys26 with Mia40 was 300-fold increased, from 0.12 s −1 to 43 s −1 ( Fig. 5a ), which is almost equal to the high rate observed for Cys36 in Cox17* ( Table 1 ). This remarkable activation completes the evidence that hydrophobic residues next to a cysteine are critically important for the rapid formation of the initial mixed disulphide between a bound substrate protein and the catalytic disulphide of Mia40. The individual cysteine residues of Cox17* differ up to 400-fold in rate when they form mixed disulphides with the mitochondrial thiol oxidase Mia40. The rates of thiol-disulphide exchange reactions are determined by three factors: the affinity for the substrate protein, the chemical reactivity of the substrate thiols and their proximity to the catalytic disulphide of Mia40 in the bound state. The initial non-covalent binding of the protein substrate to Mia40 is very important. It leads to a general, 10 4 –10 6 -fold increase in the rate of mixed disulphide formation with the cysteines of Cox17*, relative to the rate observed for the reaction with GSH, but it cannot explain the observed difference in reactivity between the individual cysteines of Cox17*. This strong difference is also not explained by variations in the intrinsic chemical reactivity of the cysteines. In the enzyme–substrate complex, the location of a particular substrate cysteine relative to the catalytic disulphide of Mia40 is critically important for its reactivity. A hydrophobic environment directs the cysteine to the non-polar groove at the active site of Mia40 and thus predisposes it for preferential reaction with the catalytic disulphide. In fact, Cys36 of Cox17 is followed by three hydrophobic residues, and therefore it reacts 400-fold more rapidly than Cys26. After the replacement of these three residues by alanines, the reactivity dropped 400-fold and Cys36 became less reactive than all other cysteines of Cox17. In a reciprocal fashion, the reactivity of Cys26 was 300-fold increased, when the three non-polar residues were placed after this cysteine. In the ‘sliding-and-docking’ model [22] , the MISS/ITS motif was suggested to direct a particular cysteine of the substrate protein to the formation of the mixed disulphide with Mia40. This motif consists of hydrophobic residues that are one and two helical turns away from the reactive cysteine. In the bound state, it is assumed that an extended native-like helix is formed already, and that the MISS/ITS residues are used specifically to orient a particular cysteine towards the catalytic disulphide bond of Mia40. In Cox17, the MISS/ITS sequence is located between the 4th and the 5th Cys, and it was proposed that the 3rd (human Cox17) or the 4th Cys (of yeast Cox17) form the initial mixed disulphide with Mia40 (ref. 22 ). Our results do not unambiguously support this model. Cys36 is remote from the MISS/ITS motif, but it formed the mixed disulphide with Mia40 more than 10-fold faster than Cys47 and Cys57 that flank this motif. We find that in the absence of MISS/ITS, binding of Cox17 to Mia40 is weakened in general, but the rate of mixed disulphide formation in the complex was only 2–5-fold decreased for Cys47, Cys57 and also for Cys36. It thus seems to exert only a minor, generic effect on mixed disulphide formation. Cox17 is a strongly polar protein ( Fig. 1d ), and sequences of more than one hydrophobic residue in a row occur at two positions only, Ile37-Leu38-Phe39 after Cys36 and Phe50-Ile51 in the MISS/ITS sequence. Apparently, these sequences are bound preferentially by Mia40 and this explains the high reactivity of Cys36 and the moderate reactivities of Cys47 and Cys57 in the enzyme–substrate complex between Mia40 and Cox17. Cys36 of Cox17 is the second cysteine of the twin CX 9 C motif. Interestingly, the three residues before and after this cysteine show a significantly higher hydrophobicity [28] than the residues surrounding the other cysteines in the mitochondrial CX 9 C proteins of yeast [29] ( Supplementary Table S2 ). The second cysteine might thus be an initial target for Mia40 in several of these proteins. When radiolabeled Cox17 variants were imported into isolated mitochondria, long-lived mixed disulphide intermediates were observed when the 3rd Cys of human Cox17 or the 4th Cys of yeast Cox17 were present, and it was concluded that these two Cys residues are essential for forming the initial mixed disulphide with Mia40 after import into the IMS [22] . However, irrespective of whether a mixed disulphide could be detected by SDS–PAGE, most of the imported Cox17 variants became oxidized and thus trapped in the IMS. Possibly, certain mixed disulphide intermediates are long-lived, not because they are formed most rapidly, but because they are trapped, as observed for Cox19 (ref. 30 ). Protein folding is often retarded by unproductive intermediates. The role of the environment of Cys36 has not been analysed in import experiments with isolated mitochondria or in binding experiments [25] . The most amino-terminal cysteines of Tim9 and Tim10 that follow the MISS/ITS motif were found in stable mixed disulphides with Mia40 after import into isolated mitochondria and hence assumed to be critically important [15] , [26] . However, yeast mutants with a substitution of this Cys by Ser are viable, similar to other Cys-to-Ser mutants in Tim9 and Tim10 (ref. 31 ). This argues against a prominent role of this cysteine adjacent to the MISS/ITS motif. The sequence analysis of all CX 9 C proteins of yeast suggested that the residues in the MISS/ITS positions are hydrophobic, because they are used to pack the helix–helix interface and thus stabilize the folded conformation of these proteins [29] . Mixed disulphide formation between Mia40 and a substrate protein starts with the formation of a non-covalent enzyme–substrate complex (Equation (1)). Mia40 shows high affinity for hydrophobic stretches that are exposed in unfolded protein chains and in folding intermediates with incomplete or incorrect disulphide bonding. It binds to unfolded forms of Cox17 within a few milliseconds, the complex is extremely dynamic and its half-life is 10–100 ms only. This is important, because it allows the complex to explore alternative binding modes by rapid dissociation and reassociation. In addition, it prevents stalling of Mia40 by the permanent binding of damaged proteins. The hydrophobic binding region of Mia40 is very close to its catalytic disulphide ( Fig. 1a,b ), and therefore cysteines adjacent to hydrophobic residues, such as Cys36 of Cox17, are predisposed for rapid mixed disulphide formation. The mixed disulphide with Cys36 would direct Cox17 towards forming the intermediate with the inner disulphide bond ( Fig. 1d,e ), which is largely unfolded and thus remains a good substrate for Mia40 for forming the second disulphide. The substrate protein must remain dynamic in the mixed disulphide with Mia40 also to allow rapid thiol-disulphide exchange. Overly strong interactions with Mia40 or the induction of premature native-like structure, such as early helix formation would interfere with further thiol-disulphide exchange. In fact, the sliding-and-docking model [22] cannot readily account for the formation of the second disulphide in CX 3 C and CX 9 C substrates of Mia40, because the hydrophobic residues of the MISS/ITS motif become buried at the helix interface during folding and are thus no longer available for Mia40 to introduce the second disulphide. To remedy this situation, it was suggested that the second disulphide forms spontaneously independent of Mia40 by reaction with GSSG or with oxygen [11] , [23] . We suggest that the hydrophobic residues of the MISS/ITS sequence are one of several targets for Mia40. Unspecific but highly dynamic binding enables Mia40 to interact with different unfolded substrates, independent of their native secondary structure, and it allows for multiple rounds of disulphide formation and isomerization. Refolding protein chains remain substrates for Mia40 as long as they expose hydrophobic surfaces. Molecules with correct disulphide bonds fold to completion and are thus no longer bound by Mia40. The decrease of hydrophobic surface thus directs the folding process. As all other folding enzymes, Mia40 does not provide specific folding information. It facilitates the folding of many different proteins, also of proteins that do not contain helices with twin CX 9 C or twin CX 3 C motifs and MISS/ITS sequences [32] , [33] , [34] . Mia40 does not belong to the thioredoxin family as all other known thiol-disulphide oxidoreductases, and unlike PDI or DsbC, it has no separate chaperone domains for substrate binding. However, it uses the same basic mechanisms for substrate binding via hydrophobic interactions, for the chemical step of mixed disulphide formation, and, possibly, for isomerizing incorrect disulphide bonds. Mia40 seems to be unique, however, in providing a hydrophobic substrate-binding site immediately adjacent to the catalytic disulphide. This enables Mia40 to direct the oxidation process by targeting cysteines in hydrophobic regions for forming the first mixed disulphide. Such cysteines often participate in buried disulphide bonds in the interior of folded proteins. They should be formed early in folding, and this might be aided by the strong preference of Mia40 for such cysteines. For simple substrates such as the CX 3 C and CX 9 C proteins with two disulphides only, this could be sufficient to warrant the correct order of disulphide formation and avoid incorrect disulphides. Materials I-AEDANS [2-iodo derivative of 5-(((acetylamino)ethyl)amino)naphthalene-1-sulphonic acid was purchased from Invitrogen (Darmstadt, Germany), sodium iodoacetate from Sigma-Aldrich (Germany). DTT, TCEP, GSH and GSSG were obtained from Roth (Karlsruhe, Germany) and GdmCl (ultra pure) from MP Biomedicals (Aurora, Ohio, USA). All other chemicals were from Roth or Grüssing (Filsum, Germany). Expression and purification of proteins Yeast Mia40 (residues 284–403) and Cox17* C16S C23S C24S were linked N terminally with the SUMO protein Smt3 from Saccharomyces cerevisiae containing an N-terminal hexahistidine tag and cloned into the expression plasmid pET11a. For Cox17 without cysteines or with the outer or inner disulphide only, we did not routinely replace cysteines by serines, as in previous work [35] . For choosing good substitute amino acids, we considered the space occupied by the cysteines in the structure of Cox17 as well as the exposure to solvent. Cys57 is exposed, and therefore it was replaced by Ser. The other cysteines are buried, and accordingly they were replaced by non-polar residues of suitable size. The burying of non hydrogen-bonded serine side chains is accompanied by a large desolvation penalty, and therefore Cys→Ser substitutions at buried position must be avoided, because they are strongly destabilizing. Cox17*-SUMO was overproduced in E . coli BL21(DE3) (Stratagene, Santa Clara, CA, USA), Mia40-SUMO in E . coli Origami B (DE3) (Novagen, Darmstadt, Germany). After lysis of the cells in 50 mM Tris–HCl, 50 mM NaCl and 10 mM EDTA, pH 8.0 and centrifugation, the SUMO-fusion proteins were obtained in a soluble form. Cox17*-SUMO was purified by immobilized metal-affinity chromatography on a 5 ml Ni-NTA column and elution with 250 mM imidazole. To avoid formation of dimers and non-native disulphides, the protein was unfolded and reduced in 0.1 M Tris–HCl, 4.0 M GdmCl, 5 mM GSH, pH 8.0 for 2 h, then diluted into refolding buffer to the final conditions of 0.1 M Tris–HCl, 0.5 mM GSH, 2 mM GSSG, pH 8.0 and incubated at room temperature overnight. The SUMO tag was cleaved with the SUMO protease SenP2 (ref. 36 ) and the SUMO fragment was removed by a second passage over the Ni-NTA column. The protein was further purified by gel filtration on a Superdex 75 prep-grade column (GE Healthcare, Uppsala, Sweden). For Cox17* variants with one cysteine only, purification was as above, but without reduction/refolding step, and the buffers contained 1 mM DTT. The reaction with Ellman's reagent [37] indicated that the single-Cys variants of Cox17* contained 0.8–1.2 equivalents of thiol groups. Crude extracts of Mia40-SUMO were incubated with Erv1 in 0.1 M Tris–HCl pH 8.0 at 4 °C for 6 h to minimize the fraction of Mia40 dimers. Further purification was performed as described for Cox17* above, but omitting the reduction/refolding step. Modification with I-AEDANS Prior to modification with I-AEDANS, Cox17* variants with single-Cys residues or Mia40/W294F/C296S were incubated with 1 mM TCEP [tris(2-carboxyethyl) phosphine hydrochloride] in 0.1 M Tris–HCl, pH 8.0, for 30 min to reduce the protein. The labelling was performed with a fivefold molar excess of I-AEDANS for Cox17* and a 1.5-fold molar excess for Mia40 for 1 h at 15 °C in the dark. The labelled protein was purified by two passages over a NAP-10 column. The extent of modification was determined by measuring the absorbance at 280 nm and 336 nm in 6.0 M GdmCl and 0.1 M potassium phosphate pH 7.4. Labelling efficiencies were generally between 95 and 105%. Reduction of Cox17* Reduced Cox17* was prepared by incubation of Cox17* variants with 50 mM DTT in 0.1 M potassium phosphate, 4.0 M GdmCl, pH 7.4 for 3 h at 25 °C. The reduced protein was purified by two passages over a NAP-10 column that had been equilibrated with nitrogen saturated buffer and then stored as a frozen solution at −80 °C. Equilibrium and kinetics of substrate association The titrations of 0.5 μM Mia40-Aedans with Cox17* F50W variants or with α-lactalbumin and 0.5 μM Cox17*-AEDANS with Mia40 were followed by the increase in the fluorescence of AEDANS at 490 nm (5 nm bandwidth) upon energy transfer from the Trp residue of Cox17* F50W variants and Mia40. Excitation was at 280 nm with a bandwidth of 3 nm. The kinetics of binding of 0.5 μM Mia40-AEDANS with Cox17* F50W variants or α-lactalbumin or 0.5 μM Cox17*-AEDANS with Mia40 were measured after stopped-flow mixing using a DX.17MV stopped-flow spectrometer from Applied Photophysics (Leatherhead, UK). The path length of the observation chamber was 2 mm. The kinetics was followed by fluorescence above 450 nm after excitation at 280 nm (10 nm bandwidth). Curves were measured at least 8 times under identical conditions, averaged and analysed as monoexponential functions. All binding experiments were performed in 0.1 M potassium phosphate, 1 mM EDTA, pH 7.4 at 15 °C. The titration curves and the profiles obtained for the binding amplitudes were analysed by assuming a 1:1 binding stoichiometry with the quadratic Equation (2) in which F is the measured fluorescence, F 0 and F ∞ are the initial and final values and [ P ] 0 and [ S ] 0 are the protein and substrate concentrations, respectively. The programme GraFit 5.0 (Erithacus Software, Staines, UK) was used for the analysis. Kinetic measurements of formation of the mixed disulphide For determination of the extent of mixed disulphide formation, 20 μM Mia40 and Cox17* variants with single-Cys residues were incubated in 0.1 M potassium phosphate, 1 mM EDTA, pH 7.4 at 15 °C. After 5 s and 5 min, respectively, the reaction was stopped by adding iodoacetate at a final concentration of 50 mM and samples were analysed by non-reducing SDS–PAGE. The kinetics of the formation of the mixed disulphide between 0.25 μM Mia40 and the single-Cys variants of Cox17* were measured after stopped-flow mixing. The kinetics was followed by fluorescence above 320 nm after excitation at 280 nm (10 nm bandwidth). Curves were measured at least 8 times under identical conditions, averaged and analysed as monoexponential functions with a linear term. Experiments were performed in 0.1 M potassium phosphate, 1 mM EDTA, pH 7.4 at 15 °C. For the determination of the apparent pK values of the cysteines in Cox17*, the kinetics of formation of mixed disulphide between 0.25 μM Mia40 and 15 μM of the single-Cys variants of Cox17* was measured as above in buffers that contained 0.1 M potassium phosphate pH 5.8, 6.2, 6.8, 7.2 and 7.4 or Tris–HCl pH 7.2, 7.4, 7.8, 8.2, 8.5 and 9. The measured rate constants were plotted against the pH value and analysed by using equation Equation (3), where k app is the apparent rate constant as derived from the fluorescence measurements and k SH and k S − are the rate constants of the reaction of the fully protonated and fully deprotonated cysteines in Cox17* with Mia40. The programme GraFit 5.0 (Erithacus Software, Staines, UK) was used for the analysis. How to cite this article : Koch, J. R. and Schmid, F. X. Mia40 targets cysteines in a hydrophobic environment to direct oxidative protein folding in mitochondria. Nat. Commun. 5:3041 doi: 10.1038/ncomms4041 (2014).